A new Argentinean nesting site showing neosauropod dinosaur reproduction in a Cretaceous hydrothermal environment Although the discoveries of fossil dinosaur eggs have exponentially increased during the last decades [1] , [2] , in situ egg clutches and nesting sites in Cretaceous exposures are still rare. Moreover, studies of these localities have largely focused on determinate factors, such as sedimentary, taxonomic or zoological observations, but the influences on the choice of these sites by sauropod dinosaurs still remained enigmatic [3] , [4] , [5] . Perhaps the most prolific and best known sauropod nesting sites are located in the Río Negro and Neuquén provinces, Argentina [5] , [6] , [7] , [8] , where the most renowned locality, Auca Mahuevo [5] , [7] , [8] , has yielded an impressive number of titanosaurid clutches [5] , [7] , [8] , [9] and eggs, some with embryos in ovo [7] , [8] , [9] , [10] . Although, this site has provided data paramount to the egg and eggshell taxonomic identification [11] , dinosaur reproductive behaviours [3] , [5] , as well as taphonomic and diagenetic processes associated with dinosaur eggs [3] , [4] , [11] , no study has addressed the underpinning factors that triggered the selection of Auca Mahuevo as a repetitive colonial nesting locality. Here, we report for the first time definitive evidences of a nesting site in a Cretaceous hydrothermal setting where a group of neosauropod dinosaurs came repetitively to ovideposit, and specifically used the soil moisture and thermoradiance to incubate their eggs at Sanagasta, La Rioja Province, Northwestern Argentina. Geology and hydrothermal settings The Sanagasta dinosaur nesting site is confined to the Cretaceous Los Llanos Formation [12] , a formation associated with the northwest Sierras Pampeanas system [12] , [13] that surfaces throughout La Rioja Province, Northwestern Argentina. Moreover, this site is restricted to the Sanagasta Valley ( Fig. 1 ). The valley comprises the Sanagasta Geologic Park (SGP, where the Sanagasta nesting site is located, La Rioja, Argentina), a 300,000 m 2 area, where Los Llanos Formation rests unconformably on red Permian sediments [12] , themselves on the lower carboniferous Sanagasta granitoid massif ( Fig. 2 ), and sub-site E, 1 km from SGP. At sub-site E, the Los Llanos formation rests directly on the Sanagasta granite ( Fig. 2 ) and is characterized by hydrothermal mega structures (30×15 m 2 and 4 m high), each of which consists of alkaline fountain geysers, vents, druses and hydrothermal pipes, all interspersed with egg clutches within 3 m from each hydrothermal relic. At SGP, the 1.5-m thick egg-bearing horizon ( Fig. 2 ) forms the upper-most section of the ( ∼ 4 m thick) Los Llanos Formation [12] , which exposes saurischian skeletons but without any oological remains and/or past hydrothermal activities in thicker outcrops ( ∼ 80 m) elsewhere in La Rioja Province. Los Llanos Formation, at SGP, is characterized by medium to coarse-grained arkosic sands (translucent, grey, whitish or yellowish colour), with low-angle tabular and trough cross-bedding interpreted as an interbraided river system [12] . Conglomerates with quartz lithoclasts are overlain by very coarse-grained sandstones cemented by calcite and silica (egg-bearing layer) with claystone intraclasts, geodes and druses of variable size with large calcite crystals ( Fig. 3a, b ; see Supplementary Fig. S1c, f, h ), thick calcareous veins ( Fig. 3c ), botryoidal siliceous structures ( Fig. 4 ; see Supplementary Fig. S2a, b ), green chrysoprase chalcedony pebbles (see Supplementary Fig. S2e ), root traces and siliceous tree trunk moulds. The Los Sauces Permian formation is vertically crosscut by calcareous and siliceous hydrothermal veins ( Supplementary Fig. S1b ), and the Cretaceous egg-bearing horizon exhibits numerous paleohydrothermal structures, mostly geysers and hot springs [14] . The lower section of the Cretaceous Los Llanos Formation displays horizontally aligned large calcite geodes and druses, typical of hydrothermal discharge channels, cavities and pipes ( Fig. 3a, b ). In addition to the stratified large horizontal veins of scalenohedron calcite crystals ( Fig. 3c ; see Supplementary Fig. S3e ), which alternates at 10 cm intervals with the arkosic sandstone ( Fig. 3c ), the upper egg-bearing level of this formation, where most of the egg clutches lay, features sedimentary structures associated with hydrothermal activities, namely, drainage and runoff of fossil mud, botryoidal quartz and chalcedonic crystals ( Fig. 4 ). These structures, which resemble the neutral environment (constructive and silica precipitation with acid overprinting) with hot spring terraces of the Yellowstone Norris Basin, are omnipresent and associated with other siliceous and calcareous structures ( Supplementary Fig. S1 ). 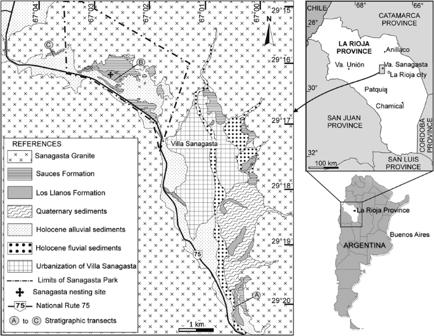Figure 1: Geographical and geological maps of Sanagasta, La Rioja Province, Argentina. (a–c) Indicates the locations of the stratigraphic profiles ofFig. 2. Figure 1: Geographical and geological maps of Sanagasta, La Rioja Province, Argentina. ( a – c ) Indicates the locations of the stratigraphic profiles of Fig. 2 . 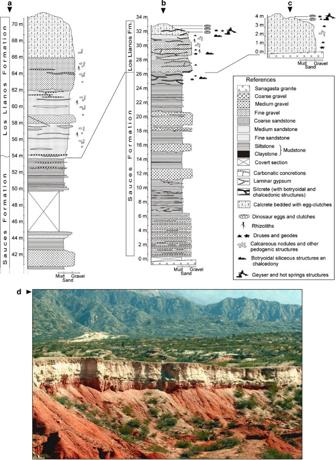Figure 2: Los Llanos Formation. Stratigraphic profile of the Cretaceous Los Llanos Formation, resting on the Sauces Formation red Lower Permian sandstones (a) outside the Sanagasta Valley. (b) Inside the Sanagasta Geological Park (SGP), where it displays both alkaline/carbonate and siliceous hydrothermal evidences; and (c) at sub-site E, outside SGP, where it directly rests on the Sanagasta granitoids and consists of hydrothermal mega structures (15 by 30 meters), interspersed with various types of vents, geyser fountains, hydrothermal conduits, and closely associated (1–3 meters) egg clutches. Only carbonate hydrothermal evidences are noted at sub-site E, akin to a Cretaceous alkaline Gondwanic Cycle geochemical composition. (d) Panoramic of SGP with the white Los Llanos Formation above the red Sauces Formation. Full size image Figure 2: Los Llanos Formation. Stratigraphic profile of the Cretaceous Los Llanos Formation, resting on the Sauces Formation red Lower Permian sandstones ( a ) outside the Sanagasta Valley. ( b ) Inside the Sanagasta Geological Park (SGP), where it displays both alkaline/carbonate and siliceous hydrothermal evidences; and ( c ) at sub-site E, outside SGP, where it directly rests on the Sanagasta granitoids and consists of hydrothermal mega structures (15 by 30 meters), interspersed with various types of vents, geyser fountains, hydrothermal conduits, and closely associated (1–3 meters) egg clutches. Only carbonate hydrothermal evidences are noted at sub-site E, akin to a Cretaceous alkaline Gondwanic Cycle geochemical composition. ( d ) Panoramic of SGP with the white Los Llanos Formation above the red Sauces Formation. 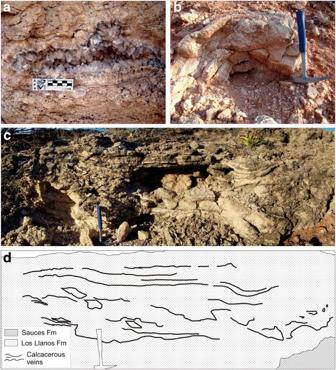Figure 3: Los Llanos Formation hydrothermal structures at SGP. (a,b) Horizontally aligned calcite geodes and druses typical of hydrothermal discharge channels, cavities and conduits. (c) Large horizontal veins of scalenohedron calcite crystals, relics of Cretaceous hydrothermal activities at SGP. (d) Schematic depiction of the calcareous veins in panelc. Full size image Figure 3: Los Llanos Formation hydrothermal structures at SGP. ( a , b ) Horizontally aligned calcite geodes and druses typical of hydrothermal discharge channels, cavities and conduits. ( c ) Large horizontal veins of scalenohedron calcite crystals, relics of Cretaceous hydrothermal activities at SGP. ( d ) Schematic depiction of the calcareous veins in panel c . 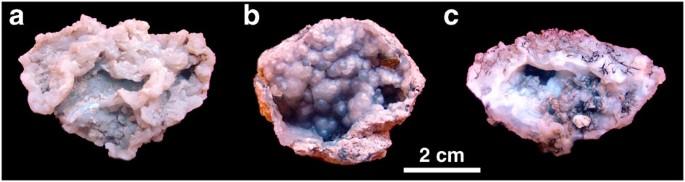Figure 4: Siliceous sinter from the nesting site. (a) White and milky cup-shaped and patchy siliceous sinter. (b) Blue and purple botryoidal chalcedonic crystals in sinter. (c) Sinter with microfacies. These ubiquitous sinters, commonly deposited by hydrothermal solutions either in deeper channels or on surface of nearby vents, add another level of support to the past hydrothermal activities that occurred in the Sanagasta Valley. Full size image Figure 4: Siliceous sinter from the nesting site. ( a ) White and milky cup-shaped and patchy siliceous sinter. ( b ) Blue and purple botryoidal chalcedonic crystals in sinter. ( c ) Sinter with microfacies. These ubiquitous sinters, commonly deposited by hydrothermal solutions either in deeper channels or on surface of nearby vents, add another level of support to the past hydrothermal activities that occurred in the Sanagasta Valley. Full size image Five hydrothermal cycles are recognized with the Sierras Pampeanas orogeny [15] , [16] . Each cycle has a distinct metallogenic and hydrothermal signature. The first three cycles predated the Mesozoic and were followed by the Cretaceous Gondwanic and tertiary Andean cycles. The former, associated with several rift basins in central-western Argentinean regions [16] , [17] , [18] , is related to the Atlantic early rifting [16] , [19] , [20] and caused the migration of moderate temperature alkaline hydrothermal solutions of low salinity but enriched with respect to F, Mn, Ba, Fe, As, Cu, Mo, Pb, V, Zn, Sr, Li, W and Sb [16] , a geochemical signature that greatly differs from that of the Tertiary Andean hydrothermal cycle. Our geochemical analyses of the Sauces and Los Llanos Formation sediments and eggshells indicate analogous concentrations with respect to the elements to the Gondwanic cycle ( Table 1 ), thus supporting a Cretaceous dating for the hydrothermal activities in the Sanagasta Valley. Table 1 Eggshell and sediment geochemical analyses. Full size table Clutches, eggs and eggshells The egg clutches rest within a 1–3 m radius from hydrothermal relics, which are abundantly distributed at 3–20 m intervals throughout the 1.5-m thick egg-bearing horizon. The spatial co-distribution of both hydrothermal evidences and egg clutches is strongly suggestive of site fidelity, colonial reproductive behaviours [5] , [7] and also synchronicity of the successive ovidepositions and ongoing hydrothermal activities during the Cretaceous period. Although most of the 80 recovered clutches contain 3–12 eggs ( Fig. 5a ), several display up to 35 eggs and extend over 1.8 m 2 with a maximum clutch axis of 220 cm. The three-dimensional geometry of the seemingly complete assemblages is well preserved and their cross-sections reveal a spatial arrangement of two superposed rows wherein the greater amount of eggs is in the upper row ( Fig. 5b ), a configuration indicating that the clutches were buried in dug-out holes rather than lying atop the soil. In addition, the high amount of eggs per clutch suggests that the Sanagasta dinosaurs ovideposited their eggs in mass, a reproductive character shared with modern crocodilians and sauropod dinosaurs [3] , [4] , [5] . The majority of the eggs are superficially fractured in multiple eggshell fragments that intricately fit together ( Fig. 5a, c ), a taphonomic pattern that implies that the eggs were complete at burial [21] , but exposed to some compression after burial when the matrix was already cemented [21] , which, in turn, limited the lateral extension of the eggshell and forced them to fracture. The mono-layered Sanagasta eggshells ( Fig. 5d, f, h, i ), which correspond to the faveoloolithid egg parataxonomic group, are characteristically thick (up to 7.94 mm) and display an exceptionally well-developed pore canal network giving them a spongy appearance ( Fig. 5f, h ). This structural characteristic is indicative of nesting environments with elevated moisture content, congruent here with the out flow of Cretaceous hydrothermal fluids. Moreover, the eggshell external surfaces exhibit rounded or subrounded to subpolygonal nodular structures ( Fig. 5e ), a biological adaptation that matches the size and sorting of the associated sediments by preventing sediments entering and blocking pore canal apertures [11] . Overall, the eggshell structural characters support a nesting environment hypersaturated with respect to moisture, which is congruent with the Sanagasta Cretaceous hydrothermal activities. 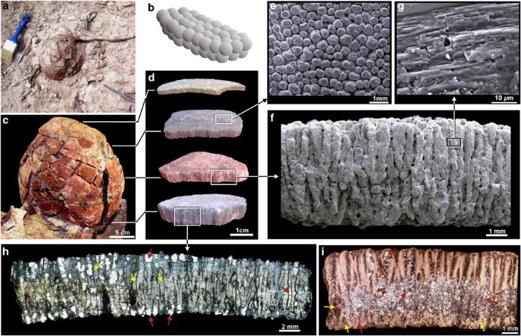Figure 5: Clutches, eggs and eggshell characteristics. (a) A 21 cm egg exposed at SGP. (b) Spatial arrangement of a complete egg clutch implying dug-out holes as 'nests'. (c) A complete egg with typical fractured eggshell. (d) Typical variation of the eggshell thickness in a single egg; (e) SEM image of outer surface of eggshells with nodes and pore apertures. (f) SEM image of radial view of eggshells. Note the spongy appearance, an adaptation to extremely wet environments. (g) Rombohedric acicular calcite crystals with vesicles. (h,i) Transmitted light microscopic views of radial section of an eggshell. Yellow arrows point to the microspar diagenetic calcite, the red arrows to the diagenetic chalcedonic crystals. Figure 5: Clutches, eggs and eggshell characteristics. ( a ) A 21 cm egg exposed at SGP. ( b ) Spatial arrangement of a complete egg clutch implying dug-out holes as 'nests'. ( c ) A complete egg with typical fractured eggshell. ( d ) Typical variation of the eggshell thickness in a single egg; ( e ) SEM image of outer surface of eggshells with nodes and pore apertures. ( f ) SEM image of radial view of eggshells. Note the spongy appearance, an adaptation to extremely wet environments. ( g ) Rombohedric acicular calcite crystals with vesicles. ( h , i ) Transmitted light microscopic views of radial section of an eggshell. Yellow arrows point to the microspar diagenetic calcite, the red arrows to the diagenetic chalcedonic crystals. Full size image Although the original eggshell calcitic structure is generally well preserved and its microstructural characters well defined, several specimens display diagenetic replacements by secondary calcite ( Fig. 5h, i ; see Supplementary Fig. S1i ), chalcedony, quartz crystals and other silicates ( Fig. 5h, i ; see Supplementary Fig. S4 and S5 ) and epidotes [12] , in moderate amounts. The large ( ∼ 21 cm diameter) Sanagasta eggs exhibit unusual thick eggshells, with a thickness variation from 1.29 to 7.94 mm, a mean of 3.847 mm, median of 4.195 mm, σ 2 =1.173 and n =307 ( Table 2 ). The thin and thick shell morphotypes, both present on the same eggs ( Fig. 5c, d ), substantiate the presence of a single ootaxon, in which the thinner eggshells reveal an outer surficial chemical dissolution often accompanied by diagenetic replacement in the eggshell units ( Fig. 5i ). Moreover, thin shells are identical to the innermost section of the thicker eggshells, and their surficial nodes resemble the outer-most surface of the weathered thicker specimens ( Fig. 5i ). Thinner eggshells display notably straight pore canals, whereas pore canals meander and coalesce in the thicker eggshell sections ( Fig. 5f ). In view of these observations, we hypothesize that the 7-mm thick eggshells ( Fig. 5a, c, d ) offered an adaptation to chemical dissolution in an extreme environment by buffering external erosion from acidic hydrothermal fluids, thus providing sufficient time for embryonic development. Table 2 Eggshell thickness variation analysis. Full size table Temperatures The presence of aluminium oxide in both eggshell and sediments ( Table 1 ), the presence of botryoidal quartz, chalcedonic crystals, chrysoprase chalcedony and associated quartz incrustations ( Fig. 4 ; see Supplementary Fig. S1 ) indicate that the temperatures of the hydrothermal solutions ranged between 60 and 190 °C [22] , [23] . Moreover, as chalcedony usually precipitates from saturated aqueous solutions at temperatures less than 100 °C [22] , [23] , [24] , [25] , [26] , this estimate could be further narrowed down to temperatures ranging from 60 to 100 °C ( Fig. 4 ; see Supplementary Fig. S1 ). According to Guidry and Chafetz [27] four different types of siliceous springs are defined in the Yellowstone Norris Basin: siliceous spires and cones, domal mounds, terraced mounds and ponds. Those with domal mounds [27] were described as discharge channels with temperatures less than 80 °C. Botryoidal silicates and domal structures formed by silicified sandstone (see Supplementary Fig. S3d ) are ubiquitous at Sanagasta and suggest the presence of a Norris-like basin epithermal environment [22] , [24] , [25] , [26] , [28] , [29] , [30] (see Supplementary Figure S6 ), with relatively low temperature (<100 °C) hydrothermal solutions that would have been sufficient to elevate and maintain soil temperatures at an adequate level to incubate 21 cm diameter eggs over a period of 1–2 months. The presence of semi-articulated skeletal remains of sauropod and theropod dinosaurs combined with the dearth of any oological or geothermal evidences in the same horizon outside SGP strongly suggest that the small and restricted Sanagasta Valley offered an ideal and exclusive setting during the Cretaceous period for a specific group of dinosaurs to lay their eggs, which belong to a unique ootaxon ( Table 2 ). No skeletal material has been yet recovered in ovo at SGP to positively identify these specimens. Therefore, until further discoveries, taxonomic identity of the parent lineage has to solely rest on comparisons with similar material from other localities, coupled with present observations of the in situ oological material. The characteristically subspherical shape of the 21-cm diameter and estimated 6,370 cm 3 eggs ( Fig. 5a, c ) point to dinosaurs larger than those from Auca Mahuevo [11] , [31] , a Cretaceous rockery with positively identified 12–14 cm titanosaurid eggs [5] , [8] , [9] , [10] , [11] . The Sanagasta eggshells display nucleation centres at their bases, rhombohedric acicular calcite crystals ( Fig. 5g ), notable nodular surficial ornamentation ( Fig. 5e ) and their thickness is considerably more than any of the other recorded extinct eggshells even those from Río Negro [6] , [32] , La Pampa [33] and South Korea [34] (see Supplementary Table S1 ). Overall, these few diagnostic features suggest a saurischian non-theropod dinosaurian parent lineage of considerable size, which coupled with the eggshell structures would indicate a sauropod [3] , [11] or more likely a neosauropod origin. Previously described oological material similar to Sanagasta has been assigned by others [6] , [12] , [32] , [33] , [35] , [36] to the faveoloolithid egg parataxonomic oogroup, which is widely distributed during the Cretaceous period and loosely associated with titanosaurid dinosaurs [32] , [33] , [35] , [36] . Although such tentative affiliation is congruent with in situ oological observations, a less inclusive neosauropod taxonomic identification would be prudent until further supportive skeletal evidences. Whether the Gondwanic hydrothermal cycle and the egg ovidepositions were coeval or not rests on the abundance of geological evidence for hydrothermal activity affecting the strata in which the nests occur. However, hydrothermally altered strata are frequently misinterpreted, because the alteration tends to obscure depositional features and often do not display the full array of characteristic features present in their modern analogues. To further complicate this situation, the Sierra Pampeanas geology is not yet fully understood and Los Llanos Formation has been alternatively considered to be Cretaceous, Miocene and reverted recently to the Cretaceous period [12] . Yet, the Gondwanic cycle is the only hydrothermal cycle dated to the Cretaceous period, in the Sierra Pampeanas. Although it is recognized to have begun ∼ 134 million years ago, its precise duration is still debated but agreed to end by the mid-Cretaceous period [16] , [17] , [18] . As mentioned above, this cycle has a typical geochemical signature that perfectly matches that of the hydrothermal sediments and eggshells found in the Sanagasta Valley, thus supporting the Cretaceous age of the Los Llanos Formation and its dinosaur eggs. Moreover, the Gondwanic cycle is known for its alkaline chemical trend [16] , [17] , which is congruent with the hydrothermal carbonate structures observed at sub-site E that rests directly on the carboniferous Sanagasta granitoid massif. At this site, outside SGP, the Cretaceous sediments, as described above, consist of longitudinal mega hydrothermal structures aligned along a east–west axis. Each structure averages 30×15 m 2 and displays several hydrothermal vents, conduits and fountain geysers interspersed throughout the 4-m thick cemented sediments that constitute the height of these mega structures. The egg clutches are always located on the same level and within an ∼ 3 m radius from individual geyser fountains, conduits and mounds throughout these mega structures. This spatial distribution is stratigraphically indicative that both the nesting and hydrothermal process were coeval and long lasting. More importantly, the correlation between clutches and hydrothermal indicators in the Sanagasta Valley and the absence of both elsewhere in the Los Llanos Formation exposures in La Rioja province further indicate that both activities were coeval and limited in space and time. Successful hatching is known to rely expressly on optimum nesting moisture content and temperatures combined with egg size and eggshell characteristics. Ground nesters such as crocodiles or several modern birds rely on specific soil conditions to insure optimal incubation. Moreover, the endemic and endangered Polynesian megapode, Megapodius pritchardii , buries its eggs at volcanically heated nesting sites in burrows with loose sediments on Niuafo Island and is solely dependent on this nesting strategy and site [37] . The evidence gathered at Sanagasta documents that a group of neosauropods must have used soil thermoradiance and moisture from a hydrothermal origin to incubate their exceptionally large eggs. Furthermore, the analytical and microscopic characterizations unlock clues in the eggshell microstructure and related sediments that respectively support a biological and environmental interdependency that favoured egg incubation by soil thermoradiance. As such, this discovery sheds lights on reproductive strategies of the Sanagasta dinosaurs, and provides the first definitive evidence for the ecologically related selection of a restricted nesting location and site fidelity behaviour by these dinosaurs. It also sheds light on the long-held question of ecological features that underpinned the choice of specific and restricted Cretaceous nesting grounds, in which neosauropod dinosaurs migrated for reproductive purposes. On the basis of this discovery, it would be parsimonious to hypothesize that other Cretaceous neosauropod reproductive sites that exhibited nesting fidelity must also have offered particular ecological settings that favoured this reproductive behaviour. Yet, whether or not the same symbiotic relationship between Sanagasta-like ecosystems and the group of neosauropods that laid their faveoloolithid eggs there existed in other faveoloolithid nesting sites needs to be explored. Eggs and eggshells Centro Regional de Investigaciones Científicas y Transferencia Tecnológica La Rioja, La Rioja Province, Argentina (CRILAR-Pv) 400 to CRILAR-Pv 409: clutches, eggs and eggshell fragments at from the Sanagasta Valley. Three and nine eggshell and sediment samples, respectively, were taken for geochemical analyses. Sediments The sediments were sampled from three different sites in the Sanagasta Valley: two from the nesting site near the egg clutches and one outside SGP. In addition, the sediments were sampled from three different levels at each site: the upper level of Sauces Formation (Lower Permian), lower Cretaceous level (3 m below the eggs) and upper Cretaceous level with clutches and eggs (see Fig. 1 ). The specimens were coded SAN 1, SAN 2 and SAN 6 (from SGP upper Permian, lower Cretaceous and upper Cretaceous, respectively); SAN 3, SAN 4 and SAN 5 (SGP upper Permian, lower Cretaceous and upper Cretaceous, respectively); SAN 7, SAN 8 and SAN 9 (outside SGP upper Permian, lower Cretaceous and upper Cretaceous, respectively). Statistical analyses Statistical analyses rest on ∼ 3,000 eggshell fragments analyzed with the STATISTICA [38] software to assess the eggshell thickness variations for the present study and future comparative work on faveoloolithid material. Petrographic thin sections For thin sections, the specimens were washed in distiled water and cut with PetroThin, dried at 40 °C in an oven for a period of 24 h, glued with compound glue (Araldit CY 248 and hardening HY 956) on glass slides of 28×48×1.8 mm 3 and thin sectioning was carried out at the (CRILAR) Petrographic Laboratory. Observations were performed with Leica DM LB light and petrographic ® DM2500 P microscopes (Leica). The images were captured with a SONY Power Had camera (SONY, 3CCD colour video camera). Scanning electron microscopy The scanning electron microscopic (SEM) analysis and preparation of the eggshell materials and image capture were performed following Grellet-Tinner's method [39] . The SEM observations were carried out with a Philips XL 30 (Philips) SEM at the Museo Argentino de Ciencias Naturales 'Bernardino Rivadavia', Buenos Aires, Argentina, Microscope Laboratory and with a LEO 1450VP SEM at the microanalysis laboratory at the Universidad Nacional de San Luís. Each specimen was mounted on aluminium stub and coated with gold or palladium. The SEM analyses were conducted at 10 kV. The samples for thin section and SEM analysis were taken from isolated eggshell fragments in egg clutches. The Leica QWin, CorelDraw X4 and Adobe Photoshop 9.0 softwares were used for storage and final processing of the images. Geochemical analyses Major and trace elements were determined at Alex Stewart (Assayers), Argentina, using ICP and ICP-OES radial lectures for elemental analyses, respectively, following the procedure ICP-AR-42/OxM code for sedimentary rock and ICP-MA-39/OxM code for eggshell samples. How to cite this article: Grellet-Tinner, G. and Fiorelli, L.E. A new Argentinean nesting site showing neosauropod dinosaur reproduction in a Cretaceous hydrothermal environment. Nat. Commun. 1:32 doi: 10.1038/ncomms1031 (2010).